The oceanic biological pump modulates the atmospheric transport of persistent organic pollutants to the Arctic Semivolatile persistent organic pollutants have the potential to reach remote environments, such as the Arctic Ocean, through atmospheric transport and deposition. Here we show that this transport of polychlorinated biphenyls to the Arctic Ocean is strongly retarded by the oceanic biological pump. A simultaneous sampling of atmospheric, seawater and plankton samples was performed in July 2007 in the Greenland Current and Atlantic sector of the Arctic Ocean. The atmospheric concentrations declined during atmospheric transport over the Greenland Current with estimated half-lives of 1–4 days. These short half-lives can be explained by the high air-to-water net diffusive flux, which is similar in magnitude to the estimated settling fluxes in the water column. Therefore, the decrease of atmospheric concentrations is due to sequestration of atmospheric polychlorinated biphenyls by enhanced air–water diffusive fluxes driven by phytoplankton uptake and organic carbon settling fluxes (biological pump). The occurrence, transport and impact of persistent organic pollutants (POPs), such as polychlorinated biphenyls (PCBs), in the Arctic Ocean (AO) has been an issue of concern due to the enhanced bioaccumulation potential of POPs in cold environments and their impact on the Arctic ecosystem and the health of human inhabitants [1] , [2] , [3] . The processes driving the transport of POPs to the AO and their occurrence have been the subject of several studies over the last two decades [1] , [2] , [3] , [4] , [5] , [6] , [7] , [8] , [9] , [10] , [11] , [12] , [13] , [14] , [15] , [16] , including the presence of POPs in the atmosphere, seawater and to a lesser extent plankton of the AO. Chemicals such as PCBs are highly hydrophobic, as measured by the octanol–water partition coefficients ( K OW ) ranging between 10 4 and 10 8 , and are semivolatile. Therefore, PCBs and other POPs can effectively undergo volatilization from primary and secondary sources, and via atmospheric transport, accumulate in aquatic organisms once deposited in the Arctic. Regardless of the multi-phase cycling and partitioning of PCBs during their transport to the Arctic, none of the previous studies performed in high-latitude oceanic regions had sampled simultaneously the gas, aerosol, seawater (dissolved and particulate) and plankton phases, nor has quantified the role of the biological pump as a control of transport of POPs to the Arctic. The biological pump is known as the process by which primary producers (phytoplankton) fix carbon dioxide, and a fraction of the new organic matter produced is exported to the deep ocean by settling particles [17] . In the context of POPs, the biological pump has been used to name the air–deep ocean transport of POPs [2] , driven by the process of accumulation of POPs in phytoplankton organic matter, which depletes the dissolved concentrations of POPs, thus enhancing the air-to-water flux of pollutants. Part of the organic matter sinks carrying POPs to deep waters [2] . While this process has received considerable attention [2] , [9] , [18] , [19] , its role as a modulator of the Arctic pollution and atmospheric transport has not been assessed in the field. In previous Arctic field studies, Sobek and Gustafsson [13] and Gioia et al . [11] reported concentration gradients of dissolved PCB in seawater off northern Europe, extending from the North Sea to off-shore waters of western Scandinavian, to Eastern Svalbard and to the ice-covered Arctic region. These authors found decreasing concentrations at higher latitudes and evidence of fractionation processes with increasing concentrations of less chlorinated PCBs at high latitudes, which are less prone to cold trapping and being sequestered by settling particles rich in organic matter (biological pump). Gas-phase concentrations have also been reported to decrease from Northern Europe to the Arctic Atlantic sector [11] , with higher concentrations near the ice-margin zone, presumably due to enhanced volatilization induced by ice melting, which could be currently enhanced due to climate change [12] . However, the North-West Atlantic Ocean, a region with dominating south west air masses carrying pollutants from industrial/population influenced areas upwind, has not been studied before in terms of PCB occurrence and cycling, and none of the previous studies reported concentrations of POPs in air, water and plankton simultaneously. Previous studies have suggested that there are several processes affecting the atmosphere-land and atmosphere-ocean exchange that may reduce the transport potential of POPs to the polar regions. These include sequestration by high organic carbon (OC) soils [20] , [21] , the role of forests as filters of POPs [22] , and based on the results of modelling studies [2] , [18] , the oceanic biological pump. Models suggest that plankton uptake and settling fluxes of organic matter reduces the atmospheric half-lives of POPs by enhancing atmospheric deposition fluxes, thus sequestering atmospheric POPs to the deep ocean. Water column biogeochemical processes are key factors driving the occurrence and settling of PCBs and other POPs in the Arctic and other oceanic regions [9] , [18] , [19] . The accumulation of hydrophobic POPs in planktonic organisms and the subsequent settling of particle- and plankton-bound PCBs have the potential to deplete dissolved-phase concentrations of POPs. The resulting enhanced air–water disequilibria of gas and dissolved-phase concentration drives a net diffusive absorption flux from the atmosphere to the water column [18] . When this happens, the atmospheric transport is strongly retarded, and even reduced, because atmospheric deposition fluxes deplete the atmospheric levels of POPs [2] . However, field evidence for the influence of the biological pump on the atmospheric occurrence and transport of POPs has not been previously reported. The objectives of the work presented here were to study the occurrence, long-range transport potential, atmospheric deposition and the role of the biological pump on the cycling of PCBs in the sub-Arctic and AO. A simultaneous sampling of atmospheric (gas and aerosol phase), seawater (dissolved and particulate phases) and plankton samples was performed in July 2007 in the Greenland Current (GC) and Atlantic sector of the AO. The gas-phase concentrations of PCBs declined during atmospheric transport over the GC with estimated half-live ranging from 1 to 4 days. The atmospheric depositional fluxes are quantified showing a high air-to-water net diffusive flux of PCBs driven by large air–water disequilibrium in their concentrations. This flux is similar in magnitude to the estimated settling flux of PCBs in the water column. The results show the first evidence from a field study of the important role that the biological pump has modulating the atmospheric transport over the ocean. The meta-analysis of the air–water disequilibrium reported in the literature for various POP families suggest that this phenomenon is generalized in high latitude/high productivity oceanic regions. Occurrence of PCBs in the GC and AO Simultaneous sampling of the atmosphere (gas and aerosol phases), seawater (dissolved and particulate phases) and plankton was carried out between Iceland and the Arctic ice-margin zone and Svalbard archipelago in July 2007 as part of the ATOS-I cruise on board R/V Hespérides . The sampling area can be divided in two different zones; the GC between Iceland and Greenland sayling flowing northeast, and the Atlantic sector of the AO ( Supplementary Fig. S1 ), as the R/V Hespérides is not an icebreaker, ice-covered regions were not sampled during the ATOS-I cruise. 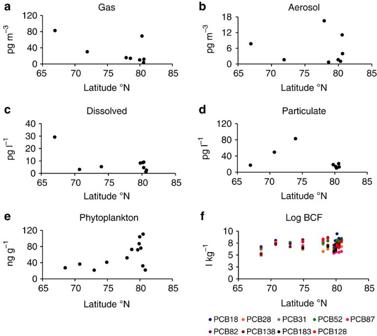Figure 1: Concentrations of polychlorinated biphenyls. PCB concentrations versus latitude in the (a) gas, (b) aerosol, (c) dissolved, (d) water particulates and (e) phytoplankton phases. Bioconcentration factor (BCF) measured for selected PCBs are shown in thefpanel. The concentrations of PCBs are the sum of congeners 18, 17, 31, 33, 52, 49, 44, 99/101, 87, 110, 82, 151, 153, 132/105, 158, 187, 183, 128, 177, 171/156, 180, 169, 201/199, 195 and 208. Figure 1 shows the latitudinal trends of PCB concentrations in the gas, aerosol, dissolved, particulate and plankton phases in the GC and AO ( Supplementary Tables S1 and S2 for individual congener concentrations). Figure 1: Concentrations of polychlorinated biphenyls. PCB concentrations versus latitude in the ( a ) gas, ( b ) aerosol, ( c ) dissolved, ( d ) water particulates and ( e ) phytoplankton phases. Bioconcentration factor (BCF) measured for selected PCBs are shown in the f panel. The concentrations of PCBs are the sum of congeners 18, 17, 31, 33, 52, 49, 44, 99/101, 87, 110, 82, 151, 153, 132/105, 158, 187, 183, 128, 177, 171/156, 180, 169, 201/199, 195 and 208. Full size image In brief, higher dissolved concentrations were found near Iceland, and lower concentrations were found near the Svalbard islands (close to the ice margin), but with some variability in this region. Dissolved PCB concentrations were well below 1 pg l −1 for most samples, consistent with other studies [11] , [13] , even though this is the first report of PCB concentrations in the GC. Particulate phase concentrations in ice-free surface seawater from the GC and AO showed considerable variability (0.01–12.29 and 0.004–9.73 pg l −1 , respectively). Finally, PCB concentrations in phytoplankton showed an increasing trend with latitude but also with a remarkable variability in concentrations close to the ice margin. Decreasing PCB concentrations during atmospheric transport The sum of total PCB concentrations (27 congeners) in the gas phase (C G ) ranged from 15.7 to 86.9 and 3.5 to 81.7 pg m −3 in the GC and AO atmospheres, respectively. The aerosol-phase concentration ranged between 1.6 to 17.3 and 0.7 to 11 pg m −3 in air over the GC and AO atmospheres, respectively. The aerosol-bound concentrations of PCBs represents on average 23% of the total atmospheric concentration due to enhanced sorption of POPs to aerosols at low temperatures. The measured gas-phase concentrations of PCBs are comparable to those reported in Bear Island (North Atlantic-Sub Arctic Region) [6] for the low chlorinated congeners, and those reported by Gioia et al . [11] for the eastern North Atlantic (3.5–22 pg m −3 for Σ 7 PCBs). The higher concentrations found by the latter in the ice-margin zone, and the climate change modulation of atmospheric POP concentrations recently described [12] , is consistent with the higher variability reported here for some congeners in the ice-margin zone, and when air masses came from coastal and ice-covered areas. The summer of 2007 holds the record for the melting of sea-ice around the North Pole [23] , which may have contributed to enhanced volatilization of POPs to the atmosphere as has been suggested recently for periods with minimum ice cover extention [12] . For some of the sampling periods (those in the GC and one close to the ice margin), the estimated air masses [24] were consistently from the southwest (North Americas origin, Supplementary Fig. S2 ). Among this subset of measurements, higher PCB concentrations were found in the southernmost sample near Iceland ( Fig. 1a , Supplementary Fig. S1 ), suggesting that atmospheric concentrations reduced during transport northwards. Indeed, measured concentrations in the gas phase showed a significant statistical decrease northwards (Friedmann test P <0.000005). The application of the Wilcoxon rank test to the data set shows that the differences of atmospheric concentrations between the sampling points are significant and establishes a gradient in the concentrations with latitude, where C G at 67°N is higher ( P <0.05) than at 74°N and significantly higher ( P <0.05) than at 78 and 81°N. It is possible to estimate the travel time ( t , days) needed for the atmospheric transport from 67°N to 81°N using the measured wind speed and wind direction ( Supplementary Table S3 ). If gas-phase concentrations are plotted against t , the atmospheric residence time ( R t ), or half-lives, can be estimated by fitting equation (1) to the measured gas-phase concentrations (see Supplementary Methods S1 for details). Where C 0 and C t are the gas concentrations near Iceland (initial) and after a time period t . R t can be related to physical–chemical properties that are relevant in the environmental partitioning of POPs, such as the octanol–water partition coefficient (log K OW ) by R t =1/(0.943 – 0.195 log K OW ) ( Fig. 2 and Supplementary Table S4 ). Examples of R t estimations are 4, 2.6 and 1.4 days for PCB congeners 18, 87 and 187, respectively. 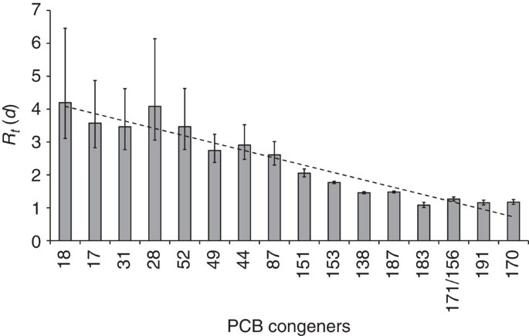Figure 2: Atmospheric residence time. Atmospheric residence times,Rt(in days), estimated for each congener using equation (1) during their transport over the Greenland Current and Arctic Ocean. Figure 2: Atmospheric residence time. Atmospheric residence times, R t (in days), estimated for each congener using equation (1) during their transport over the Greenland Current and Arctic Ocean. Full size image The estimated R t for gas-phase PCBs over the GC, ranging from 1 to 4 days ( Fig. 2 ), are consistent with those predicted in this region during the summer using a model of the atmospheric residence time of POPs [2] ( Supplementary Fig. S3 ). In the latter modelling study, the short atmospheric residence times were driven by the important role that the biological pump has enhancing the air–water exchange of PCBs in this region. Indeed, vertical settling of water column OC and associated pollutants depletes the photic zone dissolved concentrations, driving a net absorption flux of POPs from the atmosphere [2] . R t range from a few days for the less hydrophobic congeners to around 1–2 day for the more hydrophobic PCBs ( Fig. 2 ), consistent with the influence of the biological pump sequestering more effectively the more hydrophobic POPs from the atmosphere [18] . The air–deep water transport is the result of coupled air–water, phytoplankton uptake and settling fluxes [18] . The limiting step, or bottle neck, for this transfer is the diffusive air–water exchange [18] . Thus, even though the affinity to phytoplankton (or K OW ) is orders of magnitude higher for the more hydrophobic PCB congeners, the transfer of PCBs between air and deep water is limited by the air–water mass transfer coefficient that only change by a factor of 2–4 among congeners. Further support for air–water enhanced fluxes driven by the biological pump, as an explanation for the rapid decrease of atmospheric concentrations, is provided by the field measurements of dissolved, particulate and plankton concentrations and estimated air–water–plankton exchange fluxes of PCBs. Bioconcentration factors of PCBs (BCF) in plankton were estimated by [25] where C P and C W are the plankton and dissolved-phase concentrations, respectively. The study of bioconcentration of POPs, such as PCBs, in the lower levels of the trophic web is important as well to understand the factors that control the bioaccumulation and magnification of PCB concentrations in the Arctic food web, where due to the low temperatures, some POPs have longer persistence and magnification potential, leading to high concentrations in the higher predators with the associated impact on health [3] , [4] . The BCF for phytoplankton, shown in Fig. 1 , increased slightly at the northern sector of the GC, and showed higher variability near the Svalbard archipelago ( Fig. 1 ). These trends in BCF values are due in part to changes in phytoplankton community and abundance, which was dominated by colonies of Phaeocystis pouchetti , and followed by diatoms, the abundance of which showed a dependence with temperature [26] , [27] . Indeed, PCB concentrations in phytoplankton were significantly correlated with biomass abundance ( C P =2.99× Phaeocystis Biomass +43.5, r 2 =0.76, P <0.01), and the variability in seawater and plankton-phase concentrations was higher in the ice-margin zone. The influence of the ice-margin zone on the concentration of PCBs in water (and thus particle- and phytoplankton-phase concentrations) is an issue that has not been resolved. As in this study, some reports have not observed changes in water concentrations due to ice melting [11] , [26] , but the influence of ice melting on atmospheric concentrations is more conclusive [11] , [12] . A modification of gas-phase concentrations due to volatilization during ice melting has the potential to modify the seawater concentrations in proximate areas by air–water exchange inputs. The GC and Fram Strait are always regions with high phytoplankton primary productivity and chlorophyll concentrations during spring–summer. Chlorophyll a concentrations were 2.3 mg m −3 (range 0.3–6.7 mg m −3 ) [28] for the cruise stations and were high for all the GC and North Atlantic region as discerned from satellite images ( Supplementary Fig. S4 ). Primary productivity and the gross community production were also high during the sampling period [28] , [29] . Periods with high phytoplankton growth can induce lower BCF values for the more hydrophobic compounds in comparison with the BCF values for low growth conditions [25] , thus introducing further variability in the water column concentrations, consistent with the observations. Bauerfeind and co-workers [30] have shown that most sinking fluxes of OC in the Eastern Fram Strait occur during the summer (the June–September period accounts for more than 60% of the annual export of OC) and the export of OC at 300-m depth accounts for ~10% of the gross primary productivity. It is then possible to estimate the removal of PCBs associated to sinking particles using these reported summer fluxes of OC and biogenic material for the Arctic summer (May to September), and the PCB concentrations measured in particles and plankton. Thus, the settling fluxes of PCBs ( F Settling , ng per m 2 per day) are given by: Where F Biogenic is the sinking flux of biogenic material as reported elsewhere (from 35 to 40 mg per m 2 per day) [30] and C P are the PCB concentrations measured in plankton. 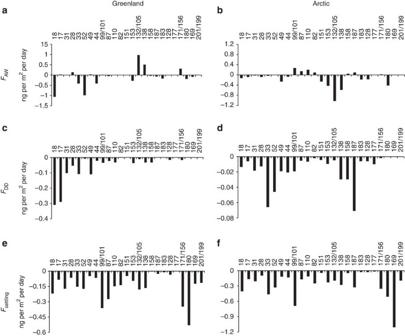Figure 3: Atmospheric deposition and settling fluxes. Net diffusive air–water exchange fluxes (FAW, ng per m2per day) for the (a) Greenland Current and (b) Arctic Ocean. Dry deposition fluxes (FDD, ng per m2per day) for the (c) Greenland Current and (d) Arctic Ocean. Settling fluxes (FSettling, ng per m2per day) of PCBs for the (e) Greenland Current and (f) Arctic Ocean. Figure 3 shows the estimated sinking fluxes for the GC and Fram Strait, respectively ( Supplementary Table S5 ). These fluxes can be compared with the atmospheric deposition fluxes of PCBs, which are the sum of net diffusive air–water exchange ( F AW ) and dry deposition ( F DD ), estimated in the traditional manner by: Figure 3: Atmospheric deposition and settling fluxes. Net diffusive air–water exchange fluxes ( F AW , ng per m 2 per day) for the ( a ) Greenland Current and ( b ) Arctic Ocean. Dry deposition fluxes ( F DD , ng per m 2 per day) for the ( c ) Greenland Current and ( d ) Arctic Ocean. Settling fluxes ( F Settling , ng per m 2 per day) of PCBs for the ( e ) Greenland Current and ( f ) Arctic Ocean. Full size image Where C G and C A are the gas- and aerosol-phase PCB concentrations, respectively, H′ is the dimensionless Henry's Law constant, k AW is the air–water mass transfer coefficient, and v D is the deposition velocity (0.1 cm s −1 ) of aerosol-bound POPs. Estimated values and details of methodology and assessment of uncertainty for the F AW and F DD can be found elsewhere [2] , [11] , [18] , [19] and in Supplementary Methods S2 . The estimated diffusive air–water exchange shows a significant net deposition of most PCB congeners in both the GC and Arctic region ( Fig. 3 and Supplementary Table S6 ). The dry deposition fluxes ( Fig. 3 and Supplementary Table S7 ) of aerosol-bound PCBs are lower than the net diffusive fluxes, but account for up to 30% of the total deposition fluxes for some congeners due to the low temperatures enhancing the sorption of PCBs to aerosols, thus increasing the dry deposition fluxes. The comparison of atmospheric deposition and sinking fluxes ( Fig. 4 ) shows that approximately the same amount of PCBs that enter the ocean from the atmosphere are settling to the deep ocean, taking into account the factor of 2–3 uncertainty in these estimations for individual compounds ( Supplementary Fig. S6 ). Therefore, the air–water–plankton–deep water system was presumably close to steady state during the sampling period with a significant coupling between the biological pump and atmospheric deposition. The high fluxes of biogenic matter during the Arctic summer depletes the water column concentrations driving a strong air-to-water fugacity gradient in the GC, which increase the diffusive flux from the atmosphere to water. This removal from the atmosphere as a depositional flux is on average of the order of 0.44 ng per m 2 per day for individual PCB congeners. A flux of this magnitude will remove an important fraction of atmospheric PCBs during their transport to the Arctic. Those PCB congeners with higher BCF values show a stronger association with phytoplankton organic matter, with higher potential for being transported to deep waters and depleting water column concentrations, thus driving a higher air–water diffusive flux. Indeed, there is a significant correlation between F AW and BCF for the data set generated in this study ( F AW =−0.15 logBCF+1.07, r 2 =0.26, P <0.05, Supplementary Fig. S5 ). 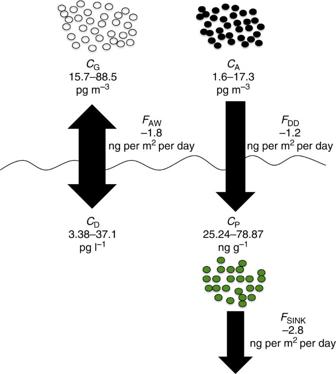Figure 4: Sequestration of PCBs in the Greenland Current. Schematics of the coupled fluxes of ΣPCBs* involved in the sequestration of atmospheric pollutants by the biological pump.CG(gas-phase concentration),CA(aerosol-phase concentration),CD(dissolved-phase concentration),CP(phytoplankton-phase concentrations),FAW(net air-to-water diffusive flux),FDD(dry deposition flux) andFSINK(settling flux). *Sum of PCBs 18, 17, 31, 33, 52, 49, 44, 99/101, 87, 110, 82, 151, 153, 132/105, 158, 187, 183, 128, 177, 171/156, 180, 169, 201/199, 195 and 208. Figure 4: Sequestration of PCBs in the Greenland Current. Schematics of the coupled fluxes of ΣPCBs* involved in the sequestration of atmospheric pollutants by the biological pump. C G (gas-phase concentration), C A (aerosol-phase concentration), C D (dissolved-phase concentration), C P (phytoplankton-phase concentrations), F AW (net air-to-water diffusive flux), F DD (dry deposition flux) and F SINK (settling flux). *Sum of PCBs 18, 17, 31, 33, 52, 49, 44, 99/101, 87, 110, 82, 151, 153, 132/105, 158, 187, 183, 128, 177, 171/156, 180, 169, 201/199, 195 and 208. Full size image The atmospheric deposition fluxes can be used to give estimates of atmospheric residence times that complement those derived from the decrease of atmospheric concentrations ( Fig. 2 ). Taking PCB congeners 153 and 180 as examples (see Supplementary Fig. S6 ), the total atmospheric concentrations (gas+aerosol) are in the range 0.9–4.7 and 1.2–4.0 pg m −3 , respectively. Considering a height of 500 m for the boundary layer, then the atmospheric inventory of PCBs 153 and 180 in the atmospheric boundary layer is 0.45–2.3 and 0.6–2.0 ng m −2 , respectively. The atmospheric residence time can be estimated by R t =inventory/net deposition [2] . The total net deposition is 0.33 and 0.2 ng per m 2 per day for PCBs 153 and 180, respectively. Then the atmospheric residence time estimated from the atmospheric concentrations (inventory) and deposition fluxes are in the ranges 1.4–7 days and 1.8–6 days for PCBs 153 and 180, respectively. These ranges of atmospheric residence times are of the same magnitude, when considering the uncertainties, than those predicted for high-chlorinated PCBs from the decrease of concentrations during atmospheric transport ( Fig. 2 ), and support the fact that the high air–water disequilibrium can account for the rapid reduction of atmospheric concentrations over productive oceans. This also suggests that the depletion of atmospheric PCBs by other processes is not relevant in comparison to atmospheric deposition. One potential candidate process might be degradation due to reaction with OH radicals, but this is negligible in this region due to low OH concentrations [2] . An important issue is whether there is remineralization of PCBs in the surface ocean, or the role that remineralization of organic matter has in the fate of PCBs and other POPs. There is no field, laboratory, nor modelling evidence of effective degradation processes for PCBs in surface seawater even in warmer regions [19] , [31] . Therefore, PCBs should be considered as persistent compounds in the oceanic water column, although sinking organic matter will be partly remineralized during sedimentation. When this happens, the fugacity capacity of the settling particles will decrease, and a fraction of PCBs will be redissolved in the meso-pelagic zone or in deep waters. Owing to sampling limitations for POPs, there are no measurements of PCBs from deep waters in the Arctic to evaluate the importance of this process. Subduction of cold surface waters has also been identified as a potential process for removing POPs from the surface ocean in the Greenland Sea [32] , but this process will only be effective regionally during winter when temperatures are low. This study provides the first field evidence of the role that the biological pump has sequestering atmospheric POPs over productive oceanic regions, and confirms that the biological pump reduces and minimizes the transport of PCBs to the Arctic during the summer. This is the first field study that reports the occurrence of PCBs in the atmosphere, seawater and plankton, simultaneously, enabling for an assessment of coupled air–water–deep water fluxes that cannot be performed with other data sets. However, the biological pump drives air and water away from equilibrium conditions for hydrophobic compounds, and thus it is possible to perform a meta-analysis of published data sets of gas and dissolved-phase concentrations of organic pollutants to further confirm the important role that the biological pump has driving a marked air–water disequilibrium in concentrations. We compiled data sets describing the gas- and dissolved-phase concentrations of organic pollutants in oceanic regions characterized by a high primary productivity and relevant for assessing the transport of POPs to the Arctic. These regions are mainly the North Atlantic and Atlantic sector of the Arctic and the regions proximate to the Bering Strait, but not the central Arctic that is covered by sea-ice, or coastal arctic regions that have land-influenced dynamics in terms of POP cycling. Fugacity (Pa) is a useful descriptor for assessing the air–water disequilibrium. The fugacity ratio of POPs between air and water ( f A /f W ) is given by, For the data set generated in this study, the fugacity ratios were higher than 3, showing an air–water disequilibrium driven by the biological pump with a significant net deposition. If this process is important at the hemispheric scale, then high fugacity ratios should have been observed in other assessments of POPs in the North Atlantic, North Pacific and the regions in the AO that show a high primary productivity. 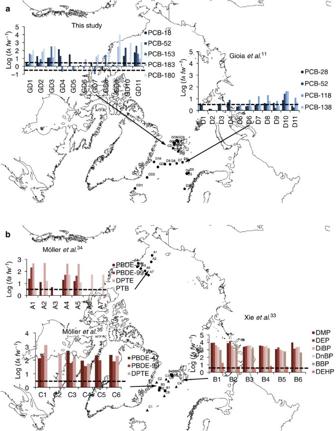Figure 5: Air–water fugacity ratios in the Arctic region. Map of the Arctic ocean, North Atlantic and North Pacific showing (a) air-to-water fugacity ratios (log(fAfW−1)) for PCBs, estimated from the gas- and dissolved-phase concentrations from this study and those reported in Gioiaet al.11and (b) air-to-water fugacity ratios (log(fAfW−1)) for other hydrophobic organic pollutants in high productivity regions from the North Atlantic and Arctic Ocean33,34,35. For all these hydrophobic chemicals, there is a strong disequilibrium between air and water (highfAfW−1) consistent with the role of the biological pump lowering water column concentrations of organic compounds. The acronyms for the chemicals stand for DMP (Dimethyl phthalate), DEP (Diethyl phthalate), DiBP (Di-i-butyl phthalate), DnBP (Di-n-butyl phthalate), BBP (n-Butylbenzyl phthalate), DEHP (Diethylhexyl phthalate), PBDE (poly-brominated diphenyl ether), PTB (pentabromotoluene), DPTE (2,3-dibromopropyl-2,4,6-tribromophenyl ether) and PCB (poly-chlorinated biphenyl). Figure 5a shows the PCB air–water fugacity ratios for this study and those reported by Gioia et al . [11] in the North Atlantic. In both cases, there is a high air–water fugacity gradient consistent with an air–water disequilibrium. Consistent with this study, Gioia et al . [11] reported higher fugacity gradients (or fluxes) for the more hydrophobic PCB congeners (higher K OW ), indicating that the biological pump has depleted the more hydrophobic compounds. Further confirmation of the role of the biological pump can be obtained from assessment of the relative abundance of the different congeners. The less hydrophobic low-chlorinated congeners are more abundant at higher latitudes [11] , [13] , a pattern that is consistent with the lower efficiency of the biological pump in removing these POPs from the water column [18] . Figure 5: Air–water fugacity ratios in the Arctic region. Map of the Arctic ocean, North Atlantic and North Pacific showing ( a ) air-to-water fugacity ratios (log( f A f W −1 )) for PCBs, estimated from the gas- and dissolved-phase concentrations from this study and those reported in Gioia et al . [11] and ( b ) air-to-water fugacity ratios (log( f A f W −1 )) for other hydrophobic organic pollutants in high productivity regions from the North Atlantic and Arctic Ocean [33] , [34] , [35] . For all these hydrophobic chemicals, there is a strong disequilibrium between air and water (high f A f W −1 ) consistent with the role of the biological pump lowering water column concentrations of organic compounds. The acronyms for the chemicals stand for DMP (Dimethyl phthalate), DEP (Diethyl phthalate), DiBP (Di- i -butyl phthalate), DnBP (Di- n -butyl phthalate), BBP ( n -Butylbenzyl phthalate), DEHP (Diethylhexyl phthalate), PBDE (poly-brominated diphenyl ether), PTB (pentabromotoluene), DPTE (2,3-dibromopropyl-2,4,6-tribromophenyl ether) and PCB (poly-chlorinated biphenyl). Full size image The biological pump may also modulate the air–water disequilibrium and atmospheric transport of other POPs than PCBs. The compilation of the few existing studies on POPs, such as phthalates [33] , polybrominated diphenyl ethers and other brominated organics [34] , [35] shows ubiquitous high air–water fugacity gradients in the high productivity regions around the AO ( Fig. 5b ). Therefore, all the field studies reporting simultaneous air and water concentrations of hydrophobic POPs show a significant disequilibrium between air and water fugacities. This further confirms the important role that the biological pump has in sequestering atmospheric POPs in the high-latitude oceanic regions, as there is no other potential mechanism that can account for these high air–water fugacity ratios. Conversely, in oligotrophic regions such as the oceanic gyres, several studies have reported volatilization of PCB in the subtropical gyres of both the south and north basins of the Atlantic and Pacific [31] , [36] , [37] , where the biological pump has a negligible role [2] , [18] . In addition, these subtropical regions are characterized by higher atmospheric degradation of PCBs due to reaction with OH radical (lowering their fugacity in the gas phase) [2] , and with warmer environments that enhances volatilization. Therefore, the modulation of atmospheric transport by the biological pump does not occur everywhere over the ocean, but only in the high productivity regions as those in high latitudes. The sequestration of atmospheric POPs by the biological pump at high latitudes is likely to be a seasonal phenomenon. Sinking fluxes of biogenic material are ten times lower during the winter [30] , thus as predicted elsewhere [2] , the atmospheric residence times during winter are expected to be much longer due to a lack of sequestration by the biological pump, with a consequent efficient transport to the AO. This will be facilitated by the fact that during the winter the Arctic atmosphere is more permeable to the Atlantic Ocean atmosphere [38] . However, transport of PCBs during the winter can not be quantified here because gas-phase concentrations in the temperate urban/industrial, rural and coastal regions upwind also depend on temperature, showing minimal concentrations during winter [39] , [40] . The temporal and geographical extent of the biological pump in northern latitudes may be modified by climate change, affecting the balance, cycling and occurrence of POPs in the AO [41] . The modulation of atmospheric transport by the biological pump is presumably also occurring in other oceanic regions globally, and both its strength and variability in space and time is currently not accounted for in models of regional/global transport of POPs. Sampling methods Air sampling was performed using a high-volume sampler (MCV: CAV-A/HF, Collbató, Spain) operating at 40 m 3 h −1 located on the upper-deck of R/V Hespérides (mean±s.e. sampled air volume 1124±381 m 3 ). The high-volume sampler was only operated when the air mass was coming from the ocean, thus avoiding potential ship contamination. This control of the ship contamination from the smokestacks was done by means of a weather vane, which interrupted the power when the air masses were from the ship sector. To sample aerosol and gas phases separately we used a precombusted (4 h at 450 °C) and preweighed Quartz Microfibre Filter (QMA 203×254 mm, 1-μm nominal pore size, Whatman, England) for the particulate phase followed by a Polyurethane Foam (PUF) plugs (100 mm diameter×120 mm, Klaus Ziemer GmbH, Germany). Both PUF and QMA filters were precleaned before the sampling. PUF was precleaned using soxhlet with Hexane/DCM (1:1) during 24 h, and QMA filters were precombusted for 4 h at 450 °C. Once the samples were taken, PUFs were packed using aluminium foil sleeves and placed into two zip-sealed bags and stored in refrigerated laboratory on board. After sampling, quartz microfibre filters were placed into aluminium foil envelopes and two zip-sealed bags, finally the aerosol samples were stored at a −20 °C fridge until sample analysis at the laboratory at Barcelona. Surface seawater (4 m depth) was sampled from an on board continuous flow system from the R/V Hespérides and transferred into an overflowing 15-l stainless steel container during the whole sampling period to avoid contamination from the ship. Seawater was pumped from this 15-l recipient with a peristaltic pump fitted with Teflon tubes through Whatman glass fibre filters (GFF, 142 mm diameter, 0.7-μm pore size) to obtain the particulate phase and through solvent-rinsed stainless steel columns, packed with XAD-2 resin (SUPELCO, USA) to obtain the dissolved phase. The XAD columns had been previously cleaned with methanol and dichloromethane and were kept in methanol at 277 K until used for sampling. Once the sample was taken (about 300 l of seawater) cartridges were resealed and placed into a refrigerated (4 °C) laboratory on board. Particulate GFF filters followed the same process, as described above, for the aerosol filters and were kept at −20 °C until analysis. Phytoplankton sampling was performed using a net trawl with a mesh size of 200 μm (RYC S.A. Girona, Spain). The net was cleaned using prefiltered seawater and unsalted water for the first time and placed into a zip-sealed bag until opening on board for sampling. The net was cleaned with abundant seawater between samples. Sampling depth was from below the maximum of chlorophyll density depth (MCD) to the surface. The time length of the tows depends on the MCD. The towing speed was 20 m min −1 from surface to MCD and 10 m min −1 from MCD to the surface. Then, the phytoplankton was filtered through a glass fibre filter (GFD, Whatman, 47 mm, 2.7-μm pore size). Copepods were removed from the sampler before filtering. GFF filters were pretreated as described for the QMA filters. Once phytoplankton samples were obtained, filters were folded, wrapped in aluminium foil, and kept in zip-sealed plastic bags in the freezer (−20 °C) until their analysis in the laboratory. All solvents used, acetone, hexane, methanol and dichloromethane, were gas chromatography quality branded (Merck, KGaA). Sample extractions and fractionation Prior to the extraction, 10 ng of PCBs 65 and 200 (PCB 65 and 200, Dr Ehrenstorfer, GmbH, Germany) were added to samples to be used as surrogates to control the analyte extraction recovery and losses during sample handling. PUFs and filters corresponding to the gas, aerosol, particulate and phytoplankton were soxhlet extracted for 24 h. For the PUF extraction acetone/hexane (3:1) was used, while hexane/dichloromethane (1:1) was used for the aerosol, particulate and phytoplankton filters. All the samples were then concentrated using a rotary evaporation unit until the sample volume was 0.5 ml. Dissolved seawater samples were extracted in eluting XAD columns using 200 ml of methanol followed by 300 ml of dichloromethane. Afterwards, the methanol fraction was liquid–liquid extracted three times with hexane. The hexane and dichloromethane fractions were merged and concentrated using rotary evaporation until the sample volume was 0.5 ml. Clean up and fractionation was done for the extracts from gas, aerosols and seawater (PUF, filters, XAD columns) using glass columns filled with neutral alumina (3 g of 3% deactivated) and anhydrous sodium sulphate (1 g). During the clean up, the sample was fractionated into three fractions. The first fraction containing the PCBs was eluted with hexane (5 ml). Finally, the hexane fraction was concentrated using a rotary evaporation, as described above, until 1–2 ml, then transferred to vials and further concentrated under a gentle N 2 stream to 150 μl and sealed. The phytoplankton samples were cleaned and fractionated using a column filled with 0.5–1 g of anhydrous sodium sulphate over 3 g of 3% deactivated neutral alumina (as described) and 5 g of silica gel (silica 60, 200 mesh) activated at 250 °C for 24 h. The first fraction was eluted using 40 ml of hexane/dichloromethane (1:2). This fraction was used to analyse concentration of PCBs in phytoplankton. More information on the analytical procedures has been described elsewhere [19] . Quantification of PCBs An Agilent 7890 coupled to a uECD detector (Agilent Technologies) using a Wcot Sil 8CB 60 m capillary column (inner diameter 0.25 mm, film thickness 0.25 μm) was used to analyse PCBs. The chromatographic programme starts from 90 °C holding for 1 min, then temperature raised from 90 to 190 °C at 20 °C min −1 and from 190 to 310 °C at 3 °C min −1 , holding 310 °C for 18 min. Retention time was used for the identification of the analytes. Internal standard quantification method was used adding 5 ng of PCBs 30 and 142 prior to injection. Compounds in the calibration standard solution were PCBs 18, 17, 31, 28, 33, 49, 44, 99/101, 87, 110, 82, 151, 153, 132/105, 138, 158, 177, 171/156, 180, 191, 169, 170 and 201/199. Quality assurance and control Detection limits (DLs) were calculated using mean plus 3 times the standard deviation of the noise in the blank samples and mean plus 10 times the standard deviation for quantification limits. The median and range of DLs for selected PCBs in different matrices are 0.015 (0.004–0.07), 0.015 (0.004–0.07), 0.007 (0.001–0.048), 0.008 (0.002–0.167) and 0.019 (0.01–0.069) ng on column for gas, aerosol, dissolved, particulate and phytoplankton, respectively. DL and quantification limit values for single PCBs are presented in Supplementary Table S10 . Statistical analysis and back trajectories Statistical analysis was performed using SPSS 19.0.0 for MacOS (SPSS, Chicago). Air mass back trajectories were estimated using the HYSPLIT transport and dispersion model from the NOAA Air Resources Laboratory ( http://www.arl.noaa.gov/ready.php ). How to cite this article: Galbán-Malagón, C. et al . The oceanic biological pump modulates the atmospheric transport of persistent organic pollutants to the Arctic. Nat. Commun. 3:862 doi: 10.1038/ncomms1858 (2012).